Histone acetylation mediated by Brd1 is crucial forCd8gene activation during early thymocyte development During T-cell development, Cd8 expression is controlled via dynamic regulation of its cis -regulatory enhancer elements. Insufficiency of enhancer activity causes variegated Cd8 expression in CD4 + CD8 + double-positive (DP) thymocytes. Brd1 is a subunit of the Hbo1 histone acetyltransferase (HAT) complex responsible for acetylation of histone H3 at lysine 14 (H3K14). Here we show that deletion of Brd1 in haematopoietic progenitors causes variegated expression of Cd8 , resulting in the appearance of CD4 + CD8 − TCRβ −/low thymocytes indistinguishable from DP thymocytes in their properties. Biochemical analysis confirms that Brd1 forms a HAT complex with Hbo1 in thymocytes. ChIP analysis demonstrates that Brd1 localizes at the known enhancers in the Cd8 genes and is responsible for acetylation at H3K14. These findings indicate that the Brd1-mediated HAT activity is crucial for efficient activation of Cd8 expression via acetylation at H3K14, which serves as an epigenetic mark that promotes the recruitment of transcription machinery to the Cd8 enhancers. During T-cell development, expression of the Cd4 and Cd8 co-receptor genes, which are required for differentiation of helper- and killer-lineage T cells, respectively, is strictly regulated. Extensive studies have proposed that stage- and lineage-specific expression of Cd8a and Cd8b1 genes is regulated by combined regulation of at least five different Cd8 enhancers (E8 I –E8 V ) in the Cd8 locus [1] . Manipulation of Cd8 enhancers in mice has unravelled the role of each enhancer in Cd8 gene regulation. Importantly, variegated expression of CD8 in double-positive (DP) thymocytes is observed in mice with combined deletion of E8 I and E8 II or deletion of E8 II and E8 III enhancers [2] , [3] , [4] . Similarly, among transcription factors implicated in the regulation of Cd8 enhancers, combined deletion of genes of Ikaros family ( Ikaros +/− Aiolos −/− ) was shown to cause variegated CD8 expression in DP thymocytes [5] . This Cd8 variegation also occurs in mice with attenuated activity of the BAF (Brahma-related gene/Brahma-associated factor) chromatin-remodelling complex. Haplo-insufficiency of Brg1, which is an ATPase required for BAF-mediated chromatin remodelling, leads to the appearance of CD8-negative DP cells, suggesting a link between Cd8 enhancers and the BAF chromatin remodelling complex [6] . Moreover, variegated CD8 expression could be partially reverted by intercrossing E8 I /E8 II doubly deficient mice with DNA methyltransferase 1 ( Dnmt1 )-deficient mice [7] . These findings suggest a link between transcription factors such as Ikaros and inhibition of DNA methylation in Cd8 gene activation. However, it remains unclear whether histone modifications are crucial for Cd8 gene activation. The histone acetyltransferases (HATs) of the MYST family include Tip60, Hbo1, Moz/Morf and Mof and function in multisubunit protein complexes. We previously reported that Bromodomain-containing protein 1 (Brd1), also known as Brpf2, forms a novel HAT complex with Hbo1 and is responsible for the global acetylation of histone H3 at lysine 14 (H3K14) [8] . However, because of embryonic lethality of Brd1 −/− mice, the function of Brd1 in regulating lymphopoiesis remains uncharacterized. In this study, we generated mice in which Brd1 is inactivated in haematopoietic progenitors and found that Brd1 plays a crucial role in the induction of CD8 expression at several stages of T-lymphocyte development. Our findings revealed that H3K14 acetylation by Brd1 is essential for efficient activation of the Cd8 gene. Deregulated T-cell development in Brd1 -deficient thymus We previously reported that Brd1 −/− mice die from severe anaemia by E13.5 or earlier [8] . To understand the role of Brd1 in adult haematopoiesis, we generated mice harbouring Brd1 fl mutation in which exon 2 containing the first ATG is floxed ( Fig. 1a ) and then crossed Brd1 fl/fl mice with Tie2-Cre mice that specifically express Cre in haematopoietic and endothelial cells ( Tie2-Cre;Brd1 fl/fl mice) [9] . Complete deletion of Brd1 in peripheral blood (PB) CD45 + mononuclear haematopoietic cells was confirmed by genomic PCR ( Supplementary Fig. 1 ). In contrast to germline deletion, which causes lethal anaemia in embryos, deletion of Brd1 in haematopoietic and endothelial cells resulted in a mild differentiation block in erythroblasts in the fetal liver, thus allowing Tie2-Cre;Brd1 fl/fl mice to be born and grow normally. 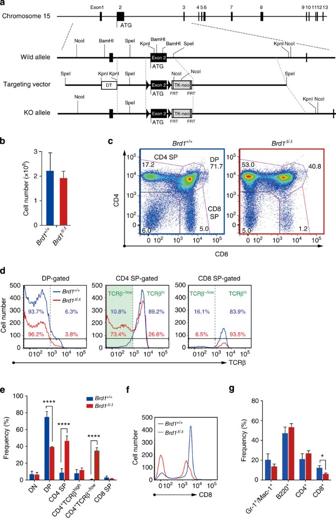Figure 1: Deregulated T-cell development in theBrd1-deficient thymus. (a) Strategy for making a conditional knockout allele forBrd1by homologous recombination in ES cells. FRT recombinase was used to remove theTK-Neocassette. (b) Absolute numbers of total thymocytes fromTie2-Cre(Brd1+/+) andTie2-Cre;Brd1fl/fl(Brd1Δ/Δ) mice. Data are presented as mean±s.d. (Brd1+/+,n=5;Brd1Δ/Δ,n=4). (c) Representative flow cytometric profiles of CD4 and CD8 expression in thymic T cells from 8- to 11-week-oldTie2-Cre(Brd1+/+) andTie2-Cre;Brd1fl/fl(Brd1Δ/Δ) mice. Proportion of each gate is indicated. (d) Representative flow cytometric profiles of TCRβ expression in DP, CD4 SP and CD8 SP cells gated in (c). Percentages of TCRβhiand TCRβ−/lowcells are shown (Brd1+/+in blue andBrd1Δ/Δin red). (e) Frequencies of indicated cell populations in total thymocytes from 8- to 11-week-oldTie2-Cre(Brd1+/+) andTie2-Cre;Brd1fl/fl(Brd1Δ/Δ) mice. Data are presented as mean±s.d. (Brd1+/+,n=5;Brd1Δ/Δ,n=4). (f) Representative flow cytometric profiles of CD8 expression in thymic T cells in (c). (g) Frequencies of myeloid (Gr-1+and/or Mac-1+), B (B220+) or T (CD4+and CD8+) cells in CD45+PB mononuclear cells from 8- to 11-week-oldTie2-Cre(Brd1+/+) andTie2-Cre;Brd1fl/fl(Brd1Δ/Δ) mice. Data are presented as mean±s.d. (Brd1+/+,n=10;Brd1Δ/Δ,n=8). *P<0.05, **P<0.01 and ***P<0.001 (Student’st-test). Figure 1: Deregulated T-cell development in the Brd1 -deficient thymus. ( a ) Strategy for making a conditional knockout allele for Brd1 by homologous recombination in ES cells. FRT recombinase was used to remove the TK-Neo cassette. ( b ) Absolute numbers of total thymocytes from Tie2-Cre ( Brd1 +/+ ) and Tie2-Cre;Brd1 fl/fl ( Brd1 Δ/Δ ) mice. Data are presented as mean±s.d. ( Brd1 +/+ , n =5; Brd1 Δ/Δ , n =4). ( c ) Representative flow cytometric profiles of CD4 and CD8 expression in thymic T cells from 8- to 11-week-old Tie2-Cre ( Brd1 +/+ ) and Tie2-Cre;Brd1 fl/fl ( Brd1 Δ/Δ ) mice. Proportion of each gate is indicated. ( d ) Representative flow cytometric profiles of TCRβ expression in DP, CD4 SP and CD8 SP cells gated in ( c ). Percentages of TCRβ hi and TCRβ −/low cells are shown ( Brd1 +/+ in blue and Brd1 Δ/Δ in red). ( e ) Frequencies of indicated cell populations in total thymocytes from 8- to 11-week-old Tie2-Cre ( Brd1 +/+ ) and Tie2-Cre;Brd1 fl/fl ( Brd1 Δ/Δ ) mice. Data are presented as mean±s.d. ( Brd1 +/+ , n =5; Brd1 Δ/Δ , n =4). ( f ) Representative flow cytometric profiles of CD8 expression in thymic T cells in ( c ). ( g ) Frequencies of myeloid (Gr-1 + and/or Mac-1 + ), B (B220 + ) or T (CD4 + and CD8 + ) cells in CD45 + PB mononuclear cells from 8- to 11-week-old Tie2-Cre ( Brd1 +/+ ) and Tie2-Cre;Brd1 fl/fl ( Brd1 Δ/Δ ) mice. Data are presented as mean±s.d. ( Brd1 +/+ , n =10; Brd1 Δ/Δ , n =8). * P <0.05, ** P <0.01 and *** P <0.001 (Student’s t -test). Full size image Detailed analysis of the lymphoid organs, however, revealed abnormal thymocyte differentiation. Although thymic cellularity of the Tie2-Cre;Brd1 fl/fl mice was comparable to that of the control mice ( Fig. 1b ), the pattern of CD4/CD8 expression was significantly altered ( Fig. 1c ). The proportion of CD4 single-positive (SP) thymocytes was significantly increased while that of DP and CD8 SP thymocytes was decreased ( Fig. 1c ). Analyses of T-cell antigen receptor (TCR) β expression revealed that a proportion of CD4 SP thymocytes of Tie2-Cre;Brd1 fl/fl mice expressed no or low levels of TCRβ (TCRβ −/low ) like control DP thymocytes ( Fig. 1d ). DP thymocytes in Tie2-Cre;Brd1 fl/fl mice were reduced twofold compared with the control mice. Instead, the CD4 + TCRβ −/low thymocytes were found at a frequency comparable to that of DP thymocytes in Tie2-Cre;Brd1 fl/fl mice ( Fig. 1e ). In contrast, the frequency of bona fide CD4 + TCRβ high SP thymocytes in Tie2-Cre;Brd1 fl/fl mice was comparable to that of the control mice ( Fig. 1e ). Interestingly, the level of CD8 expression in Brd1 Δ/Δ thymocytes was moderately but significantly lower than that of the control, with the mean fluorescent intensity (MFI) of DP and CD8 SP thymocytes in flow cytometric analysis being 66.1% and 80.8% of the control, respectively ( Fig. 1f ). To better distinguish mature from immature thymocytes and reveal their CD4 and CD8 coreceptor expression patterns in Tie2-Cre;Brd1 fl/fl mice, we fractionated thymocytes for their expression of TCRβ and CD69 ( Supplementary Fig. 2 ). As expected, WT TCRβ − CD69 − thymocytes were mostly CD4 + CD8 + DP thymocytes, whereas Brd1 Δ/Δ thymocytes contained a large number of CD4 SP cells along with DP cells, suggesting that the large portion of CD4 SP cells are at a similar differentiation stage to DP thymocytes. Of interest, a significant portion of Brd1 Δ/Δ mature TCRβ + CD69 + and TCRβ + CD69 − thymocytes appeared as CD4 −/low CD8 − subset. This result may reflect that some MHC class I-selected thymocytes during maturation towards the CD8 lineage are unable to express CD8 ( Supplementary Fig. 2 ). In addition, CD4 −/low CD8 − cells were detected also in the immature TCRβ − CD69 − fraction, suggesting that failure of Cd8 gene activation at the transition from DN to DP stage in the absence of Brd1 allows a significant portion of Brd1 Δ/Δ DN cells to differentiate into CD4 + TCRβ −/low thymocytes directly via CD4 low TCRβ −/low intermediate stage ( Supplementary Fig. 2 ). We next analysed mature T-cell pools in the periphery, and found that the frequency of mature CD8 + T cells in PB was decreased to 50% of the control ( Fig. 1g and Supplementary Fig. 3 ). All CD4 + T cells showed a high level of TCRβ expression and no CD4 + CD8 − TCR −/low T cells were detected in the PB of Tie2-Cre;Brd1 fl/fl mice ( Supplementary Fig. 3 ). Among TCRβ + cells, however, there was a mild increase in the population of CD4 − CD8 − cells in the PB of Tie2-Cre;Brd1 fl/fl mice compared with the controls. It is possible that some class I-restricted cells in the PB are phenotypically CD8 − CD4 − due to the compromised expression of CD8 ( Supplementary Fig. 3 ). Cell autonomous defect of T cells in the absence of Brd1 The Tie2 promoter drives Cre expression not only in haematopoietic cells, but also in endothelial cells [9] . To exclude any influence of loss of Brd1 on the thymic microenvironment, we transplanted BM cells from Tie2-Cre control and Tie2-Cre;Brd1 fl/fl mice (CD45.2 + ) with the same number of BM competitor cells (CD45.1 + ) into lethally irradiated wild-type recipient mice (CD45.1 + ). Recipient mice reconstituted with Brd1 Δ/Δ BM cells showed abnormal thymocyte differentiation similar to that in the Tie2-Cre;Brd1 fl/fl mice ( Fig. 2a,b ). Brd1 Δ/Δ T cells were markedly outcompeted by the T cells derived from the competitor cells in the PB ( Fig. 2c ). We therefore transplanted BM cells from Tie2-Cre;Brd1 fl/fl mice without competitor cells and again found that Brd1 Δ/Δ T cells, particularly CD8 + T cells, were outcompeted by the residual host T cells ( Fig. 2d ). These results indicate that the appearance of abnormal CD4 + CD8 − TCRβ −/low thymocytes and the inefficient production of mature CD8 + T cells are intrinsic to Brd1 Δ/Δ cells. 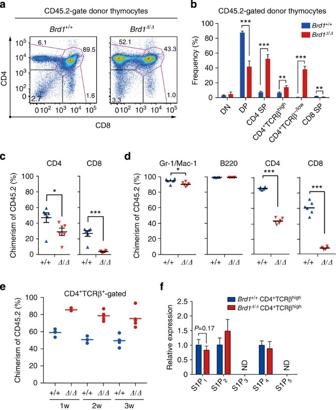Figure 2: Cell autonomous defect of T cells in the absence of Brd1. (a) Surface expression of CD4 and CD8 onBrd1Δ/Δcells in recipient mice. BM cells fromTie2-Crecontrol (Brd1+/+) andTie2-Cre;Brd1fl/fl(Brd1Δ/Δ) mice (CD45.2+) were transplanted into lethally irradiated wild-type recipient mice (CD45.1+) along with the same number of BM competitor cells (CD45.1+). Representative flow cytometric profiles of CD4 and CD8 expression in CD45.2+donor-derived T cells in the thymus at 6 months post-transplantation are depicted. The proportion of each gate is indicated. (b) Frequencies of indicated cell populations in CD45.2+donor-derived T cells in (a). Data are presented as mean±s.d. (Brd1+/+,n=5;Brd1Δ/Δ,n=5). (c) Contribution ofBrd1Δ/Δhaematopoietic cells to the PB T lymphocytes of recipient mice in (a). Chimerism of donor-derived CD45.2+Brd1Δ/Δcells in the PB at 12 weeks post-transplantation is shown as mean±s.d. (Brd1+/+,n=6;Brd1Δ/Δ,n=6). (d) Contribution ofBrd1Δ/Δhaematopoietic cells to the PB in recipient mice. BM cells fromTie2-Crecontrol (Brd1+/+) andTie2-Cre;Brd1fl/flmice (Brd1Δ/Δ) (CD45.2+) were transplanted into lethally irradiated wild-type recipient mice (CD45.1+) without any BM competitor cells. Chimerism of donor-derived CD45.2+Brd1Δ/Δcells in the PB at 12 weeks post-transplantation is shown as mean±s.d. (Brd1+/+,n=6;Brd1Δ/Δ,n=6). (e) Competitive repopulating capacity ofBrd1Δ/Δperipheral CD4 T cells. CD4 T cells from theTie2-Crecontrol andTie2-Cre;Brd1fl/flspleen (1 × 106each, CD45.2) were transferred into sublethally irradiated NOG mice along with the same number of CD45.1 splenic CD4 T cells (competitor cells). Chimerism of CD45.2+Brd1Δ/ΔCD4 T cells in the PB CD4+TCRβ+T-cell pool is plotted as dots and mean values are indicated as bars. (f) Expression of S1P receptors inBrd1Δ/ΔCD4+TCRβhighthymocytes. Quantitative RT-PCR analysis of the expression of S1P receptor genes inBrd1+/+andBrd1Δ/ΔCD4+TCRβhighthymocytes was performed.Hprt1was used to normalize the amount of input RNA. ND=not detected. *P<0.05, **P<0.01 and ***P<0.001 (Student’st-test). Figure 2: Cell autonomous defect of T cells in the absence of Brd1. ( a ) Surface expression of CD4 and CD8 on Brd1 Δ/Δ cells in recipient mice. BM cells from Tie2-Cre control ( Brd1 +/+ ) and Tie2-Cre;Brd1 fl/fl ( Brd1 Δ/Δ ) mice (CD45.2 + ) were transplanted into lethally irradiated wild-type recipient mice (CD45.1 + ) along with the same number of BM competitor cells (CD45.1 + ). Representative flow cytometric profiles of CD4 and CD8 expression in CD45.2 + donor-derived T cells in the thymus at 6 months post-transplantation are depicted. The proportion of each gate is indicated. ( b ) Frequencies of indicated cell populations in CD45.2 + donor-derived T cells in ( a ). Data are presented as mean±s.d. ( Brd1 +/+ , n =5; Brd1 Δ/Δ , n =5). ( c ) Contribution of Brd1 Δ/Δ haematopoietic cells to the PB T lymphocytes of recipient mice in ( a ). Chimerism of donor-derived CD45.2 + Brd1 Δ/Δ cells in the PB at 12 weeks post-transplantation is shown as mean±s.d. ( Brd1 +/+ , n =6; Brd1 Δ/Δ , n =6). ( d ) Contribution of Brd1 Δ/Δ haematopoietic cells to the PB in recipient mice. BM cells from Tie2-Cre control ( Brd1 +/+ ) and Tie2-Cre;Brd1 fl/fl mice ( Brd1 Δ/Δ ) (CD45.2 + ) were transplanted into lethally irradiated wild-type recipient mice (CD45.1 + ) without any BM competitor cells. Chimerism of donor-derived CD45.2 + Brd1 Δ/Δ cells in the PB at 12 weeks post-transplantation is shown as mean±s.d. ( Brd1 +/+ , n =6; Brd1 Δ/Δ , n =6). ( e ) Competitive repopulating capacity of Brd1 Δ/Δ peripheral CD4 T cells. CD4 T cells from the Tie2-Cre control and Tie2-Cre;Brd1 fl/fl spleen (1 × 10 6 each, CD45.2) were transferred into sublethally irradiated NOG mice along with the same number of CD45.1 splenic CD4 T cells (competitor cells). Chimerism of CD45.2 + Brd1 Δ/Δ CD4 T cells in the PB CD4 + TCRβ + T-cell pool is plotted as dots and mean values are indicated as bars. ( f ) Expression of S1P receptors in Brd1 Δ/Δ CD4 + TCRβ high thymocytes. Quantitative RT-PCR analysis of the expression of S1P receptor genes in Brd1 +/+ and Brd1 Δ/Δ CD4 + TCRβ high thymocytes was performed. Hprt1 was used to normalize the amount of input RNA. ND=not detected. * P <0.05, ** P <0.01 and *** P <0.001 (Student’s t -test). Full size image Given the essential requirement for CD8 as a co-receptor to support the differentiation of CD8 T cells, it is likely that the low CD8 expression in the thymus is causal for the reduction of CD8 T cells. However, Brd1 Δ/Δ CD4 T cells also showed significantly lower chimerism in PB in competitive repopulation experiments ( Fig. 2d ). We therefore tested the ability of Brd1 Δ/Δ peripheral CD4 T cells to repopulate in immunocompromised host mice. We transferred 1 × 10 6 CD45.2 CD4 T cells from the Tie2-Cre control and the Tie2-Cre;Brd1 fl/fl spleen into sublethally irradiated NOG mice along with the same number of CD45.1 splenic CD4 T cells (competitor cells). Brd1 Δ/Δ CD4 T cells established chimerism that is comparable to or rather higher than that of the control cells ( Fig. 2e ). Considering that the number of Brd1 Δ/Δ CD4 + TCRβ high SP thymocytes is comparable to that of the WT control, these results suggest that the reduced chimerism of Brd1 Δ/Δ CD4 T cells in the periphery could be attributed to the impaired egress from the thymus to the periphery. To test this hypothesis, we checked the expression of S1P receptors (S1P 1–5 ), which regulate the egress of T cells from the thymus [10] . Although expression of S1P 1 , which is critical for CD4 SP thymocytes to egress from the thymus [10] , showed a trend of reduction in Brd1 Δ/Δ CD4 + TCRβ high thymocytes, it did not give a statistical significance ( Fig. 2f ). These findings suggest that Brd1 is necessary to endow appropriate integrity to CD4 T cells in the periphery. We then examined whether Brd1 was required for CD4 T-cell function. We purified splenic naive CD4 T cells from WT and Tie2-Cre;Brd1 fl/fl mice and cultured them under Th1 or Th2 conditions in vitro . Intriguingly, the numbers of both IFNγ-producing cells under Th1 conditions and IL-4-producing cells under Th2 conditions were decreased substantially by loss of Brd1 ( Supplementary Fig. 4 ). These findings indicate that Brd1 is also required for efficient cytokine production by peripheral CD4 T cells. Variegated Cd8 expression in the absence of Brd1 We next characterized the cell cycle status of Brd1 Δ/Δ CD4 + CD8 − TCRβ −/low thymocytes reconstituted in wild-type thymic environment using a BrdU incorporation assay. Both control and Brd1 Δ/Δ DP thymocytes contained a significant proportion of cycling cells, whereas CD4 + CD8 − TCRβ high and CD8 SP thymocytes did not ( Fig. 3a ). Of note, Brd1 Δ/Δ CD4 + CD8 − TCRβ −/low thymocytes contained cycling cells at the same frequency as DP thymocytes. 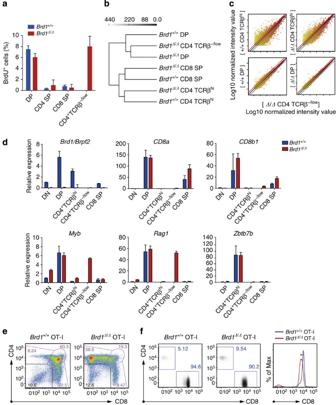Figure 3: Inefficient activation ofCd8genes inBrd1-deficient DP thymocytes. (a) Cell cycle status of repopulated thymocytes. Percentages of cells in S phase in the indicated populations of thymocytes from the recipient mice inFig. 2dwere measured by detecting incorporated BrdU by flow cytometry at 2 h post-intraperitoneal injection of BrdU. Data are presented as mean±s.d. (Brd1+/+,n=4;Brd1Δ/Δ,n=3). (b) Hierarchical clustering of gene expression patterns of the indicated cell fractions obtained in microarray analyses. For clustering analysis, the Ward’s linkage rule was applied to all expressed genes in each of the sorted cells. The Ward’s linkage scores are indicated on the top. (c) A scatter diagram of microarray analysis. The average signal levels of indicated cell fractions compared with those ofBrd1Δ/ΔCD4+CD8−TCRβ−/lowcells are plotted. The upper and lower lines represent the borderline for a twofold increase and a twofold decrease, respectively. (d) Quantitative RT-PCR analysis of the expression of the genes indicated inBrd1+/+andBrd1Δ/Δthymocytes.Hprt1was used to normalize the amount of input RNA. (e) Representative flow cytometric profiles of CD4 and CD8 expression in thymic T cells from 8- to 11-week-oldTie2-Cre(Brd1+/+) andTie2-Cre;Brd1fl/fl(Brd1Δ/Δ) mice expressing OT-I TCR transgene. Proportion of each gate is indicated. Data are representative of three independent experiments. (f) Representative flow cytometric profiles of CD4 and CD8 expression in PB ofBrd1+/+OT-I andBrd1Δ/ΔOT-I mice (left panels). Proportion of each gate is indicated. CD8 expression in PB T cells is also depicted in histograms (right panel). Figure 3: Inefficient activation of Cd8 genes in Brd1 -deficient DP thymocytes. ( a ) Cell cycle status of repopulated thymocytes. Percentages of cells in S phase in the indicated populations of thymocytes from the recipient mice in Fig. 2d were measured by detecting incorporated BrdU by flow cytometry at 2 h post-intraperitoneal injection of BrdU. Data are presented as mean±s.d. ( Brd1 +/+ , n =4; Brd1 Δ/Δ , n =3). ( b ) Hierarchical clustering of gene expression patterns of the indicated cell fractions obtained in microarray analyses. For clustering analysis, the Ward’s linkage rule was applied to all expressed genes in each of the sorted cells. The Ward’s linkage scores are indicated on the top. ( c ) A scatter diagram of microarray analysis. The average signal levels of indicated cell fractions compared with those of Brd1 Δ/Δ CD4 + CD8 − TCRβ −/low cells are plotted. The upper and lower lines represent the borderline for a twofold increase and a twofold decrease, respectively. ( d ) Quantitative RT-PCR analysis of the expression of the genes indicated in Brd1 +/+ and Brd1 Δ/Δ thymocytes. Hprt1 was used to normalize the amount of input RNA. ( e ) Representative flow cytometric profiles of CD4 and CD8 expression in thymic T cells from 8- to 11-week-old Tie2-Cre ( Brd1 +/+ ) and Tie2-Cre;Brd1 fl/fl ( Brd1 Δ/Δ ) mice expressing OT-I TCR transgene. Proportion of each gate is indicated. Data are representative of three independent experiments. ( f ) Representative flow cytometric profiles of CD4 and CD8 expression in PB of Brd1 +/+ OT-I and Brd1 Δ/Δ OT-I mice (left panels). Proportion of each gate is indicated. CD8 expression in PB T cells is also depicted in histograms (right panel). Full size image Furthermore, hierarchical clustering of gene expression profile in several thymocyte fractions from Brd1 +/+ and Brd1 Δ/Δ mice revealed that Brd1 Δ/Δ CD4 + CD8 − TCRβ −/low thymocytes have an expression profile highly similar to DP thymocytes, particularly to Brd1 Δ/Δ DP thymocytes, but quite different from mature (TCRβ hi ) CD4 SP thymocytes of both Brd1 +/+ and Brd1 Δ/Δ genotypes ( Fig. 3b,c ). Quantitative RT-PCR confirmed that Brd1 Δ/Δ CD4 + CD8 − TCRβ −/low thymocytes express genes specific to DP thymocytes, such as Myb and Rag1 (refs 11 , 12 ), but not Cd8a and Cd8b1 ( Fig. 3d and Supplementary Table 1 ). Expression of key regulator genes of Cd8 transcription, such as Ikaros , Runx1 and Runx3 , was not altered in Brd1 Δ/Δ DP and CD4 + CD8 − TCRβ −/low thymocytes compared with that in WT DP thymocytes ( Supplementary Table 1 ). These results indicate that Brd1 Δ/Δ CD4 + CD8 − TCRβ −/low thymocytes correspond to immature thymocytes that would normally appear as DP thymocytes. Correspondingly, expression of Zbtb7b that encodes Th-POK, a master regulator of CD4 helper T cells, was not detected in Brd1 Δ/Δ CD4 + CD8 − TCRβ −/low thymocytes as was not detected in WT DP thymocytes. However, its expression in Brd1 Δ/Δ CD4 + CD8 − TCRβ high thymocytes was comparable to that in WT CD4 SP thymocytes ( Fig. 3d ). To investigate whether the lack of Brd1 affects the direction of class I-restricted thymocytes to CD8 SP cells, we crossed Tie2-Cre;Brd1 fl/fl mice with mice expressing OT-I MHC class I-restricted transgenic TCR [13] . As expected, the vast majority of Brd1 Δ/Δ DP thymocytes appeared as CD8 − DP (CD4 + CD8 − TCRβ −/low ) thymocytes ( Fig. 3e ). However, some of the canonical Brd1 Δ/Δ DP thymocytes were positively selected and differentiated into mature CD8 SP thymocytes. In the PB, CD8 + T cells dominated even in the absence of Brd1, although they exhibited a reduced level of CD8 expression ( Fig. 3f ). On the basis of these findings, we conclude that Brd1 deficiency causes variegated expression of CD8 due to inefficient activation of the Cd8 gene. Of interest, expression of Brd1 is upregulated during transition of DN to DP stage and is downregulated afterwards ( Fig. 3d ). Thus, it is possible that an increase in the amount of Brd1 is necessary to initiate Cd8 activation during the DN to DP transition. To test this notion, we cultured DN3 cells on TSt-4/DLL stromal cells and monitored their differentiation. As clearly demonstrated in Fig. 4 , the majority of Brd1 Δ/Δ DN3 cells differentiated into CD4 + CD8 − TCRβ −/low thymocytes without going through the CD4 + CD8 + DP stage. These findings well correspond to the in vivo finding that a small but significant subpopulation of TCRβ − CD69 − immature thymocytes exhibits a CD4 −/low CD8 − phenotype in the Tie2-Cre;Brd1 fl/fl thymus ( Fig. 1c and Supplementary Fig. 2 ). 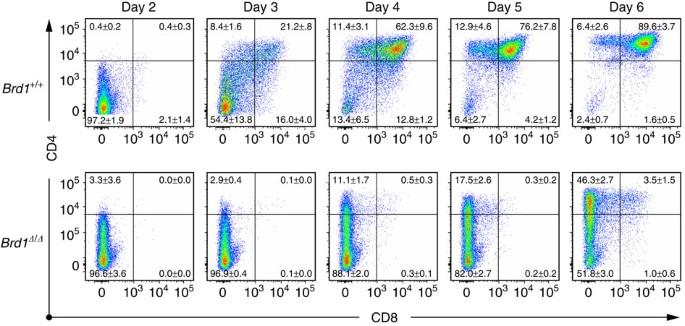Figure 4:In vitrodifferentiation ofBrd1Δ/ΔDN3 cells. DN3 cells fromTie2-Crecontrol (Brd1+/+) andTie2-Cre;Brd1fl/fl(Brd1Δ/Δ) mice were seeded on TSt-4/DLL stromal cells in triplicate and their differentiation was monitored. Cytokines (10 ng ml−1SCF, IL-7 and Flt3L) were supplemented only for the initial 24 h. Representative CD4 and CD8 expression profiles from the three repeated experiments are depicted. The proportion of each gate is indicated. Figure 4: In vitro differentiation of Brd1 Δ/Δ DN3 cells. DN3 cells from Tie2-Cre control ( Brd1 +/+ ) and Tie2-Cre;Brd1 fl/fl ( Brd1 Δ/Δ ) mice were seeded on TSt-4/DLL stromal cells in triplicate and their differentiation was monitored. Cytokines (10 ng ml −1 SCF, IL-7 and Flt3L) were supplemented only for the initial 24 h. Representative CD4 and CD8 expression profiles from the three repeated experiments are depicted. The proportion of each gate is indicated. Full size image We next examined the apoptotic status of Brd1 Δ/Δ CD8 SP thymocytes with lower CD8 expression and found that they do not show any enhancement in apoptotic cell death compared with the control cells (Annexin V + cells; Brd1 +/+ 8.4%, n =2 versus Brd1 Δ/Δ 6.1%, n =2). Impaired reactivation of Cd8 in Brd1 Δ/Δ peripheral T cells In the gut intraepithelial lymphocyte (IEL) compartment, there are three cell subsets expressing the Cd8a gene other than conventional CD8αβ + cytotoxic T cells; γδT cells, CD8αα + and CD4 + CD8αα + αβT cells [14] . We therefore examined CD8 expression in those cells. Of interest, the population of CD8αα + and CD4 + CD8αα + αβT cells were significantly decreased in Tie2-Cre;Brd1 fl/fl mice compared with the Tie2-Cre control mice ( Fig. 5 ). In addition, the percentage of CD8αα expressing γδT cells was significantly reduced ( Fig. 5 ). We interpreted the reduction in CD8αα + γδT cells as a reflection of variegated CD8 expression in γδT cells in the gut. It has also been reported that CD4 + CD8αα + IELs are differentiated from CD4 + T cells by reactivating the Cd8a gene after the downregulation of Th-POK, a master regulator of CD4 helper T cells [15] . Together, these findings suggest that Brd1 is required to initiate Cd8a activation in γδT cells as well as Cd8 reactivation in CD4 + T cells in the gut. 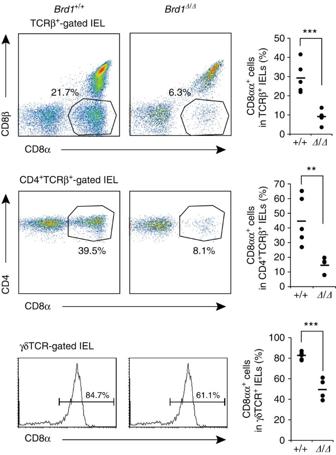Figure 5: Impaired CD8 expression in IEL subsets in the absence of Brd1. Expression of CD8αα in TCRβ+, CD4+TCRβ+and γδTCR+IELs was analysed inTie2-Crecontrol (Brd1+/+) andTie2-Cre;Brd1fl/fl(Brd1Δ/Δ) mice. Representative flow cytometric profiles from the two repeated experiments with a proportion of each gate (left panels) and the percentages of CD8αα+cells in the indicated cell populations with mean values (right panels) are shown. **P<0.01 and ***P<0.001 (Student’st-test). Figure 5: Impaired CD8 expression in IEL subsets in the absence of Brd1. Expression of CD8αα in TCRβ + , CD4 + TCRβ + and γ δ TCR + IELs was analysed in Tie2-Cre control ( Brd1 +/+ ) and Tie2-Cre;Brd1 fl/fl ( Brd1 Δ/Δ ) mice. Representative flow cytometric profiles from the two repeated experiments with a proportion of each gate (left panels) and the percentages of CD8αα + cells in the indicated cell populations with mean values (right panels) are shown. ** P <0.01 and *** P <0.001 (Student’s t -test). Full size image Brd1-Hbo1 complex is responsible for H3K14 acetylation at Cd8 gene loci To confirm that Brd1 acts as a histone modifier, we compared levels of histone acetylation between Tie2-Cre and Tie2-Cre;Brd1 fl/fl thymi. As we reported previously in Brd1 −/− erythroblasts [8] , the global level of H3K14 acetylation was profoundly decreased in Brd1 Δ/Δ thymocytes, whereas the levels of H3K9, H4K5, K8, K12 and K16 were not significantly changed ( Fig. 6a ). Biochemical analysis also confirmed that Brd1 forms a HAT complex with Hbo1 and Ing4/5 in the AKR1 DP T cell line expressing 3xFlag-Brd1 (AKR1/Brd1 cells) ( Supplementary Fig. 5 ). Chromatin immunoprecipitation (ChIP) assays of AKR1/Brd1 and AKR1/Hbo1 cells confirmed that Brd1 and Hbo1 bind to the enhancers and promoters of the Cd8 genes, respectively ( Fig. 6b ). ChIP assays also revealed drastic reduction in levels of H3K14 acetylation at the enhancers and promoters of the Cd8a and Cd8b1 loci in Brd1 Δ/Δ DP thymocytes and even more reduction in Brd1 Δ/Δ CD8 − DP thymocytes. In contrast, the reduction was only moderate at the Cd4 silencer in both Brd1 Δ/Δ DP and CD8 − DP thymocytes, which express CD4 ( Fig. 6b ). These findings suggest that the Hbo1-Brd1 HAT complex acetylates H3K14 at the transcriptional regulatory elements of the Cd8 gene, and that this step is necessary for efficient activation of the Cd8 gene. 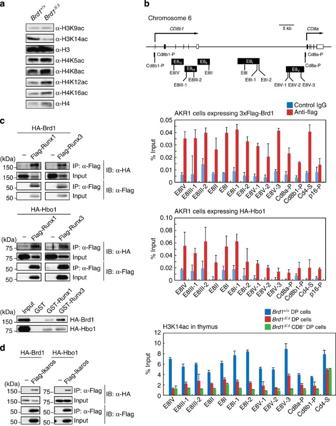Figure 6: Brd1-Hbo1 complex acetylates H3K14 at theCd8gene loci. (a) Levels of acetylation at histone H3 and H4 in total thymocytes fromTie2-Cre(Brd1+/+) andTie2-Cre;Brd1fl/fl(Brd1Δ/Δ) thymus. Histones purified from thymocytes were analysed by western blotting using the indicated antibodies. (b) Levels of H3K14 acetylation at the enhancers and promoters of theCd8aandCd8b1genes. Schematic representation of theCd8aandCd8b1gene loci and the location of the primer sets are depicted (upper panel). The binding of Brd1 and Hbo1 to theCd8aandCd8b1gene loci was determined by ChIP using an anti-Flag antibody in AKR1/3 × Flag-Brd1 cells and anti-HA antibody in AKR1/HA-Hbo1 cells, respectively. The relative amount of immunoprecipitated DNA is depicted as a percentage of input DNA. An isotype control IgG was used as a negative control. TheCd4silencer element andp16promoter served as controls. The data are shown as the mean±s.d. for triplicate PCRs (middle panel). ChIP analyses were performed usingBrd1+/+andBrd1Δ/ΔDP cells andBrd1Δ/ΔCD4+CD8−TCRβ−/lowcells purified by cell sorting and an anti-acetylated H3K14 antibody. The relative amount of immunoprecipitated DNA is depicted as a percentage of input DNA. TheCd4silencer element served as a control. The data are shown as the mean±s.d. for triplicate PCRs (lower panel). (c) Brd1 and Hbo1 directly interact with Runx proteins. 293T cells were transfected with Flag-tagged Runx1 or Runx3 together with either HA-tagged Brd1 or Hbo1. Runx proteins were immunoprecipitated using an anti-Flag antibody, and then immunoprecipitates were detected by immunoblotting using anti-Flag and anti-HA antibodies (upper and middle panels). The direct interactions between Runx proteins with Brd1 and Hbo1 were confirmed by GST-pull down assays using GST-Runx1 and GST-Runx3 fusion proteins andin vitrotranslated HA-tagged Brd1 and Hbo1 following immunoblotting using an anti-HA antibody (lower panels). (d) Brd1 and Hbo1 directly interact with Ikaros proteins. 293T cells were transfected with Flag-tagged Ikaros together with either HA-tagged Brd1 or Hbo1. Ikaros protein was immunoprecipitated using an anti-Flag antibody, and then immunoprecipitates were detected by immunoblotting using anti-Flag and anti-HA antibodies. Figure 6: Brd1-Hbo1 complex acetylates H3K14 at the Cd8 gene loci. ( a ) Levels of acetylation at histone H3 and H4 in total thymocytes from Tie2-Cre ( Brd1 +/+ ) and Tie2-Cre;Brd1 fl/fl ( Brd1 Δ/Δ ) thymus. Histones purified from thymocytes were analysed by western blotting using the indicated antibodies. ( b ) Levels of H3K14 acetylation at the enhancers and promoters of the Cd8a and Cd8b1 genes. Schematic representation of the Cd8a and Cd8b1 gene loci and the location of the primer sets are depicted (upper panel). The binding of Brd1 and Hbo1 to the Cd8a and Cd8b1 gene loci was determined by ChIP using an anti-Flag antibody in AKR1/3 × Flag-Brd1 cells and anti-HA antibody in AKR1/HA-Hbo1 cells, respectively. The relative amount of immunoprecipitated DNA is depicted as a percentage of input DNA. An isotype control IgG was used as a negative control. The Cd4 silencer element and p16 promoter served as controls. The data are shown as the mean±s.d. for triplicate PCRs (middle panel). ChIP analyses were performed using Brd1 +/+ and Brd1 Δ/Δ DP cells and Brd1 Δ/Δ CD4 + CD8 − TCRβ −/low cells purified by cell sorting and an anti-acetylated H3K14 antibody. The relative amount of immunoprecipitated DNA is depicted as a percentage of input DNA. The Cd4 silencer element served as a control. The data are shown as the mean±s.d. for triplicate PCRs (lower panel). ( c ) Brd1 and Hbo1 directly interact with Runx proteins. 293T cells were transfected with Flag-tagged Runx1 or Runx3 together with either HA-tagged Brd1 or Hbo1. Runx proteins were immunoprecipitated using an anti-Flag antibody, and then immunoprecipitates were detected by immunoblotting using anti-Flag and anti-HA antibodies (upper and middle panels). The direct interactions between Runx proteins with Brd1 and Hbo1 were confirmed by GST-pull down assays using GST-Runx1 and GST-Runx3 fusion proteins and in vitro translated HA-tagged Brd1 and Hbo1 following immunoblotting using an anti-HA antibody (lower panels). ( d ) Brd1 and Hbo1 directly interact with Ikaros proteins. 293T cells were transfected with Flag-tagged Ikaros together with either HA-tagged Brd1 or Hbo1. Ikaros protein was immunoprecipitated using an anti-Flag antibody, and then immunoprecipitates were detected by immunoblotting using anti-Flag and anti-HA antibodies. Full size image HATs are known to collaborate with the transcription factors critical for the transcriptional activation of the given genes. We therefore searched for physical interactions between the Hbo1-Brd1 HAT with Runx family transcription factors and Ikaros, which are known critical regulators that activate the Cd8 genes [5] , [16] . To identify physical interactions, we co-transfected 293T cells with Runx1 or Runx3 together with either Brd1 or Hbo1 and performed immunoprecipitation. Both Brd1 and Hbo1 were readily co-immunoprecipitated with Runx1 and Runx3 ( Fig. 6c ). These direct interactions were confirmed by GST-pull down assays using GST-Runx1 and GST-Runx3 and in vitro translated Brd1 and Hbo1 ( Fig. 6c ). We also detected co-immunoprecipitation of Ikaros with Brd1 or Hbo1 in 293T cells in a similar transfection assay ( Fig. 6d ). These results support the idea of crosstalk between transcription factors and the Hbo1-Brd1 HAT complex in the activation of Cd8 genes. Finally, to confirm the role of Brd1 in the initial activation of Cd8 gene, we transduced Brd1 Δ/Δ DN cells with a Brd1 retrovirus and cultured them on TSt-4/DLL stromal cells. Defective CD8 expression on differentiating Brd1 Δ/Δ DN cells was completely rescued by exogenous Brd1, allowing Brd1 Δ/Δ DN cells to become DP cells in vitro ( Fig. 7a ). Corresponding to this finding, the global level of acetylation at H3K14 in DP cells was largely restored by retroviral complementation of Brd1 ( Fig. 7b ). These results confirm the critical role of the acetylation at H3K14 by the Hbo1-Brd1 HAT complex in the transcriptional activation of Cd8 gene. 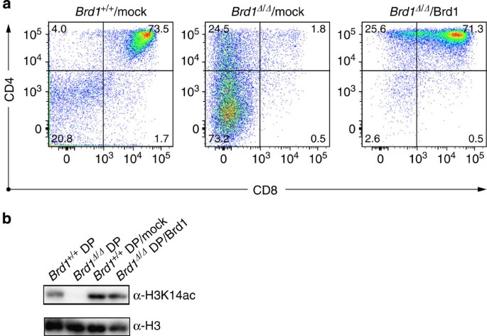Figure 7:In vitrodifferentiation ofBrd1Δ/ΔDN3 cells. (a) DN3 thymocytes fromTie2-Cre;Brd1fl/fl(Brd1Δ/Δ) mice were seeded on TSt-4/DLL stromal cells in the presence of 10 ng/ ml−1SCF, IL-7 and Flt3L and transduced with aBrd1retrovirus. At day 3 post-transduction, transduced GFP+cells were purified by cell sorting and further cultured on TSt-4/DLL stromal cells in the presence of 2 ng ml−1SCF, IL-7 and Flt3L for 7 to 10 days. DN3 thymocytes fromTie2-Cre(Brd1+/+) andTie2-Cre;Brd1fl/fl(Brd1Δ/Δ) mice without transduction served as controls. Representative CD4 and CD8 expression profiles from three repeated experiments are depicted. The proportion of each gate is indicated. (b) Levels of acetylation at H3K14 in rescued DP cells. DP cells were derived fromBrd1-transducedBrd1Δ/ΔDN1/2 thymocytes (Brd1Δ/ΔDP/Brd1, lane 4) and from WT DN1/2 thymocytes (Brd1+/+DP/mock, lane 3) as in (a) and were subjected to western blotting using an anti-H3K14ac antibody (left panel). DP thymocytes fromTie2-Cre(Brd1+/+DP, lane 1) andTie2-Cre;Brd1fl/fl(Brd1Δ/ΔDP, lane 2) thymus served as controls. Figure 7: In vitro differentiation of Brd1 Δ/Δ DN3 cells. ( a ) DN3 thymocytes from Tie2-Cre;Brd1 fl/fl ( Brd1 Δ/Δ ) mice were seeded on TSt-4/DLL stromal cells in the presence of 10 ng/ ml −1 SCF, IL-7 and Flt3L and transduced with a Brd1 retrovirus. At day 3 post-transduction, transduced GFP + cells were purified by cell sorting and further cultured on TSt-4/DLL stromal cells in the presence of 2 ng ml −1 SCF, IL-7 and Flt3L for 7 to 10 days. DN3 thymocytes from Tie2-Cre ( Brd1 +/+ ) and Tie2-Cre;Brd1 fl/fl ( Brd1 Δ/Δ ) mice without transduction served as controls. Representative CD4 and CD8 expression profiles from three repeated experiments are depicted. The proportion of each gate is indicated. ( b ) Levels of acetylation at H3K14 in rescued DP cells. DP cells were derived from Brd1 -transduced Brd1 Δ/Δ DN1/2 thymocytes ( Brd1 Δ/Δ DP/Brd1, lane 4) and from WT DN1/2 thymocytes ( Brd1 +/+ DP/mock, lane 3) as in ( a ) and were subjected to western blotting using an anti-H3K14ac antibody (left panel). DP thymocytes from Tie2-Cre ( Brd1 +/+ DP, lane 1) and Tie2-Cre;Brd1 fl/fl ( Brd1 Δ/Δ DP, lane 2) thymus served as controls. Full size image In this study, variegated expression of CD8 was observed in Brd1 Δ/Δ DP thymocytes in a manner similar to DP thymocytes with insufficient activity of Cd8 enhancers [2] , [3] , [4] . Several molecules have been implicated in the regulation of Cd8 enhancers, including Ikaros and Runx family transcription factors [5] , [16] , BAF chromatin-remodelling complex [6] and Dnmt1 [7] . However, the role of histone modifications has never been characterized before. N-terminal tail domains of histones are acetylated in the promoter region of actively transcribed genes [17] . Acetyl-lysine residues are recognized by bromodomain-containing factors. Although the role of acetylation at H3K14 is not well understood, it has been reported that several bromodomain-containing proteins such as BAF57, a subunit of the BAF chromatin remodelling complex, and TAFII250, which recruits TFIID, bind to acetylated H3K14 (refs 18 , 19 ). Indeed, compromised BAF activity causes variegated CD8 expression in a manner similar to that caused by the loss of Brd1, suggesting a functional crosstalk between the Hbo1-Brd1 HAT complex and the BAF complex [6] . It is therefore possible that the Hbo1-Brd1 complex is involved in the chromatin relaxation via H3K14 acetylation, which is followed by subsequent recruitment of transcriptional complexes at the Cd8 enhancers for full activation of the Cd8 locus. Although the expression of CD8 on the cell surface was moderately decreased in Brd1 Δ/Δ DP and CD8 SP thymocytes and Brd1 Δ/Δ CD8 + T cells in the PB, mRNA expression of Cd8a and Cd8b1 genes in these CD8 expressing Brd1 Δ/Δ cells was comparable to that of the control cells. These results suggest that the Hbo1-Brd1 HAT complex and presumably acetylation at H3K14 are required in the initiation of Cd8 transcription at the transition of DN to DP stage, but once the Cd8 transcription is activated by the compensatory action of other HATs, it can be maintained even in the absence of Brd1. Nevertheless, failure of CD8αα induction in CD4 T cells in the gut indicates that Brd1 is required to reactivate Cd8 transcription even in the peripheral T cells. These findings highlight the role of the Hbo1-Brd1 HAT complex in the activation but not the maintenance of Cd8 expression. Of note, Brd1 Δ/Δ CD4 T cells also showed significantly lower chimerism in PB, although the capacity of Brd1 Δ/Δ peripheral CD4 T cells to repopulate in immunocompromised host mice was almost intact. We therefore suspected that the reduced chimerism of Brd1 Δ/Δ CD4 T cells in the periphery could be attributed to the impaired egress from the thymus to the periphery. Indeed, the expression of S1P 1 , which is critical for CD4 SP thymocytes to egress from the thymus, showed a mild, albeit not statistically significant, reduction in Brd1 Δ/Δ CD4 + TCRβ high thymocytes, suggesting a moderate defect of Brd1 Δ/Δ CD4 SP thymocytes in egression into the periphery. In addition, given the substantial difference in gene expression profiles between WT and Brd1 Δ/Δ peripheral CD4 T cells ( Fig. 3b ), Brd1 could also be necessary to endow appropriate integrity to CD4 SP thymocytes during terminal differentiation process. Furthermore, Brd1 Δ/Δ peripheral CD4 T cells were demonstrated to be defective in producing cytokines. Together, all these findings implicate Brd1 in various aspects of the immune cell development and functions. Advances in epigenetic research are revealing the fine epigenetic regulations that control developmentally regulated gene expression, including those involved in haemato-lymphopoiesis [20] , [21] . Our findings in this study provide novel insights into epigenetic control of T-cell development. Characterization of the crosstalk between the Hbo1-Brd1 HAT complex and other regulators would promote the understanding of the complex regulation of the co-receptor expression, an essential step in the development of thymocytes. Mice and gene targeting of Brd1 For conditional deletion of Brd1 , the targeting vector was designed as in Fig. 1 , and Brd1 fl/fl mice were generated using R1 embryonic stem (ES) cells according to the conventional protocol. Brd1 fl/fl mice were backcrossed to the C57BL/6 background more than seven times and crossed with Tie2-Cre mice [9] . Eight-week-old female C57BL/6 (CD45.2) mice were purchased from Japan SLC. Eight-week-old female C57BL/6 mice congenic for the Ly5 locus (CD45.1) were purchased from Sankyo-Lab Service Corporation. OT-I mice (C57BL/6) were purchased from the Jackson Laboratory. Mice were bred and maintained in the Animal Research Facility of the Graduate School of Medicine, Chiba University in accordance with institutional guidelines. Flow cytometry and antibodies The mAbs were purchased from BD Biosciences, eBioscience or BioLegend. For analysis of co-receptor expression in adult thymocytes, cells were stained with CD45.2-PacificBlue (1:200, 104), CD4-APC (1:50, GK1.5), CD8α-PE (1:25, 53–6.7) and TCRβ chain-APC/Cy7 (1:50, H57–597). For fetal DN thymocytes, cells were stained with CD3ε-Brilliant Violet (1:50, 145–2C11), CD4-Biotin (1:50, GK1.5), CD8-APC/Cy7 (1:50, 53–6.7), CD25-APC (1:50, PC61), CD44-PE (1:50, IM7) and CD69-PE/Cy7 (1:50, H1.2F3). A biotin-labelled CD4 antibody was visualized with Streptavidin (1:50, PE/Cy7). For cell cycle analysis, incorporated BrdU was measured by using APC BrdU Flow Kit (BD Biosciences) according to the manufacturer’s protocol on gated DP, CD4 SP, CD4 + CD8 − TCRβ −/low and CD8 SP cells. For PB cells, CD45.1-PE/Cy7 (1:50, A20), CD45.2-FITC (1:50, 104), B220-APC (1:50, RA3–6B2), Gr-1-PE (1:200, RB6–8C5), Mac-1-PE (1:200, M1/70), CD4-APC/Cy7 or -APC (1:50, RM4–5 or 1:50, GK1.5) and CD8α-APC/Cy7 or -PE (1:50, 53-6.7) were used. Other antibodies used are γδTCR-biotin (1:50, GL3), NK1.1 (PK136), CD11c (N418), CD25-APC (1:50, PC61) and CD44-PE (1:50, IM7). Dead cells were eliminated by staining with propidium iodide (1 μg ml −1 ; Sigma-Aldrich). For Annexin V staining, cells were suspended with 1xAnnexin binding buffer and stained with FITC-Annexin V following the manufacturer’s protocol (BD Biosciences). All flow cytometric analyses and cell sorting were performed on FACSAria II or FACSCanto II (BD Biosciences). IELs were isolated as previously described [22] . DN3 culture Using a biotinylated lineage mixture [Gr-1, Mac-1, Ter-119, B220 (1:40), CD4, CD8α (1:10), γ Δ TCR, CD3ε, CD11c and NK1.1 (1:20)], CD25-APC(1:50, PC61) and CD44-PE(1:50, IM7), Lin − CD25 + CD44 + DN3 thymocytes were sorted on a FACSAria II. DN3 cells were cultured on TSt-4/DLL stromal cells with 10 ng ml −1 SCF, IL-7 and Flt3L (Peprotech) supplemented only for the initial 24 h. For rescue experiments, Brd1 Δ/Δ DN1/2 or DN3 cells were transduced with a Brd1 retrovirus (pMC-3xFlag-Brd1-IRES-EGFP [8] ) on TSt-4/DLL stromal cells. Transduced GFP + cells were purified by cell sorting and then cultured as described above. Competitive repopulating assay of peripheral CD4 T cells We transferred 1 × 10 6 CD45.2 CD4 T cells purified from the Tie2-Cre control and Tie2-Cre;Brd1 fl/fl spleen into sublethally irradiated NOG mice (2.0 Gy) along with the same number of CD45.1 splenic CD4 T cells (competitor cells). Chimerism of CD45.1 competitor CD4 T cells and CD45.2 test CD4 T cells in the PB was monitored weekly. Induction of Th1 and Th2 cytokine expression CD4 + T cells with a naive phenotype (CD4 + CD62L hi ) were purified with a FACSAria cell sorter (Becton Dickinson), which yielded a purity of >98%, and were used as naive CD4 + T cells. Naive CD4 + T cells (1.5 × 10 6 ) were stimulated for 2 days with immobilized mAb to TCRβ (10 μg ml −1 ; H57-597) plus soluble mAb to CD28 (1 μg ml −1 ; 37.51; BioLegend) in the presence of IL-2 (15 ng ml −1 ), IL-12 (10 ng ml −1 ; Wako) and mAb to IL-4 (5 μg ml −1 ; 11B11) for Th1 conditions, or in the presence of IL-2 (15 ng ml −1 ), IL-4 (100 ng ml −1 ; PeproTech) and mAb to IFN-γ (5 μg ml −1 ; R4-6A2) for Th2 conditions. Cells were cultured for an additional 4 days without stimulation of the TCR in the presence of the original cytokines. Cultured cells were restimulated for 6 h with immobilized mAb to TCRβ (10 μg ml −1 ), and intracellular staining was done as described [23] . BM transplantation BM cells from B6-CD45.2 mutant mice (test cells) were transplanted intravenously into 8-week-old B6-CD45.1 recipients irradiated at a dose of 9.5 Gy with or without BM cells from 8-week-old B6-CD45.1 congenic mice (competitor cells). Immunoprecipitation and GST pull-down assay 293T cells were transfected with pcDNA3-Flag-human Runx1, human Runx3 or mouse Ikaros together with either pcDNA3-HA-mouse Brd1 or mouse Hbo1. The cells were lysed in lysis buffer containing 250 mM NaCl and then immunoprecipitation was performed using anti-FLAG M2 affinity gel. Immunocomplexes were eluted with FLAG peptide. Histone proteins were extracted following the method described previously [24] . For GST pull-down assays, DNA fragments encoding the full-length human Runx1 and Runx3 were subcloned into the pGEX6p vector. GST fusion proteins were expressed in BL21 (DE3) cells. For the GST pull-down assay, HA-tagged Brd1 or Hbo1 was translated in vitro using a TNT reticulocyte lysate transcription/translation system (Promega) and mixed with GST-fusion proteins. The reaction was carried out in lysis buffer containing 150 mM NaCl at 4 °C for 2 h and the beads were washed four times with the same buffer. Proteins were separated by sodium dodecyl sulfate–PAGE (SDS–PAGE), transferred to a PVDF membrane and detected by western blotting using the following antibodies at a 1:1,000 dilution except for anti-histone H3 (1:2,000): anti-FLAG (clone M2; Sigma), anti-HA (clone 3F10; Roche), anti-HA (rabbit IgG, Santa Cruz), anti-acetyl-histone H3 (lys9), anti-acetyl-histone H3 (lys14), anti-histone H3 (rabbit IgG; Millipore), anti-acetyl-histone H4 (lys5) (clone EP1000Y), anti-acetyl-histone H4 (lys8), anti-acetyl-histone H4 (lys12), anti-acetyl-histone H4 (lys16) and anti-histone H4 (rabbit IgG; Millipore). Uncropped raw scans of blots used in the figures are presented in Supplementary Figs 6–8 . Microarray analysis Gene expression profiles were evaluated using the Agilent one-colour microarray-based gene expression platform according to the manufacturer’s instructions (Low Input Quick Amp Labeling). Total RNA (10 ng) was amplified and labelled using the one-colour Quick Amp labeling kit (51900612; Agilent Technologies). Complementary RNA (cRNA) samples were hybridized onto SurePrint G3 Mouse GE 8 × 60 K Microarray (G4852A, Agilent Technologies). The microarray numerical values were analysed using the GeneSpring GX 11.5.1 software (Agilent Technologies). For clustering analysis, the Ward’s linkage rule was applied to all expressed genes in each sorted cells. Microarray and ChIP-sequence data were deposited in Gene Expression Omnibus (accession number GSE48797). qRT-PCR Total RNA was isolated using TRIZOL LS solution (Invitrogen) and reverse-transcribed by the ThermoScript RT-PCR system (Invitrogen) with an oligo-dT primer or random hexamers. Real-time quantitative RT-PCR (qRT-PCR) was performed with an ABI Prism 7300 Thermal Cycler (Applied Biosystems) using SYBR Premix Ex TaqII (TaKaRa) and primers listed in Supplementary Table 2 . Chromatin immunoprecipitation assay AKR1 DP T cells expressing 3 × Flag-Brd1 (AKR1/Brd1 cells) or HA-Hbo1 (AKR1/Hbo1 cells) were prepared. Primary thymocytes and AKR1 cells were crosslinked with 1% formaldehyde for 5–10 min at 37 °C, washed two times with W&B buffer (100 mM Na Phosphate (pH7.0) and 0.1% Tween 20), and lysed with RIPA buffer (10 mM Tris (pH 8.0), 140 mM NaCl, 1 mM EDTA, 1% TritonX-100, 0.1% SDS, 0.1% Sodium deoxycholate (DOC) and protease inhibitor cocktail) and sonicated 15 times for 20 s using a Bioruptor (Cosmo Bio). The average chromatin fragment size after sonication was ~200–300 bp. After centrifugation, the soluble chromatin fraction was recovered, precleared for 1 h at 4 °C with a mixture of Protein A and G-conjugated Dynabeads (Invitrogen) blocked with BSA and salmon sperm DNA (Invitrogen), and then incubated with an anti-Flag, an anti-HA or an anti-acetyl H3K14 antibody (07–449; Millipore) for 2 h at 4 °C. Chromatin was immunoprecipitated overnight at 4 °C with antibody-conjugated Dynabeads. The immunoprecipitates were extensively washed with the following combination of wash buffers; RIPA buffer (10 mM Tris (pH 8.0), 150 mM NaCl, 1 mM EDTA, 1% TritonX-100, 0.1% SDS, 0.1% DOC and protease inhibitor cocktail), high salt (500 mM NaCl) RIPA buffer, LiCl wash buffer (10 mM Tris–HCl (pH 8.0), 250 mM LiCl, 1 mM EDTA, 0.5% NP40 and 0.5% DOC) and TE buffer (10 mM Tris–HCl (pH 8.0) and 1 mM EDTA). Bound chromatin and input DNA were placed in elution buffer (10 mM Tris–HCl (pH 8.0), 5 mM EDTA, 300 mM NaCl and 0.5% SDS) and reverse crosslinked. Immunoprecipitated DNA and input DNA were treated with RNase A (Sigma-Aldrich) and proteinase K (Roche). To separate DNA from protein fragments, phenol-chloroform is used in conjunction with a standard DNA purification method. For ChIP assay, quantitative PCR was performed with an ABI prism Step One Plus real time PCR system using SYBR Premix Ex Taq II (Takara Bio). The primer sequences are listed in Supplementary Table 2 . Statistical analysis Statistical tests were carried out using Graph Pad Prism version 6. How to cite this article: Mishima, Y. et al. Histone acetylation mediated by Brd1 is crucial for Cd8 gene activation during early thymocyte development. Nat. Commun. 5:5872 doi: 10.1038/ncomms6872 (2014).